Fast nanomechanical spectroscopy of soft matter A method that combines high spatial resolution, quantitative and non-destructive mapping of surfaces and interfaces is a long standing goal in nanoscale microscopy. The method would facilitate the development of hybrid devices and materials made up of nanostructures of different properties. Here we develop a multifrequency force microscopy method that enables simultaneous mapping of nanomechanical spectra of soft matter surfaces with nanoscale spatial resolution. The properties include the Young’s modulus and the viscous or damping coefficients. In addition, it provides the peak force and the indentation. The method does not limit the data acquisition speed nor the spatial resolution of the force microscope. It is non-invasive and minimizes the influence of the tip radius on the measurements. The same tip is used to measure in air heterogeneous interfaces with near four orders of magnitude variations in the elastic modulus, from 1 MPa to 3 GPa. Non-invasive, label-free and high-resolution methods for imaging surfaces and interfaces that provide simultaneous information about different material properties are needed to understand heterogeneous interfaces and to develop materials with tailored properties at the nanoscale. In fact, the evolution of the atomic force microscope (AFM) is being shaped by the need to provide a full and non-invasive characterization of complex interfaces such as solid–liquid interfaces [1] , [2] , [3] , [4] , heterogeneous polymer interfaces [5] , [6] , [7] , energy-storage devices [8] , cells [9] , [10] or protein membranes [11] , [12] , [13] , [14] . Ideally, those methods should complement the high spatial resolution of AFM with the following properties: (1) material characterization independent of the probe properties; (2) quantitative; (3) minimal tip and sample preparation; and (4) compatible with high-speed data acquisition and imaging. In the recent years, several methods have been proposed to complement the high spatial resolution of the force microscope with quantitative information about the mechanical properties of the interface [15] , [16] , [17] , [18] , [19] , [20] , [21] , [22] , [23] , [24] , [25] , [26] , [27] , [28] , [29] , [30] , [31] , [32] , [33] , [34] . In fact, the goal of combining topography with compositional contrast can be traced back to the origin of dynamic AFM with the development of phase-imaging AFM. However, there are two major differences between phase-imaging AFM [35] , [36] and the novel nanomechanical spectroscopy approaches. In nanomechanical spectroscopy, the emphasis rests in the connection between the experimental observables and the properties of the material (surface). The measurements have to be quantitative so that in the lower spatial resolution limit they could be compared with the values given by macroscale measurements. The nanomechanical information that a force microscope can obtain from a surface includes elastic and dissipative components. Elastic component, as well as some dissipative components such as adhesion hysteresis, are contained in the force measured in quasistatic equilibrium, as a function of the tip-surface separation (force curve) [37] . To determine non-conservative or velocity-dependent components, a dynamic measurement of the force is required. The combination of acquiring force curves at a single point of the surface with AFM imaging is usually known as force volume images [37] . This approach has been very successful and is widely used in combination with several contact and near-contact AFM imaging configurations [12] , [26] ; however, it has some limitations. First, the sensitivity of the force curve depends on the cantilever force constant. Thus, it might be hard to use the same cantilever for measuring heterogeneous surfaces, especially if the material has large variations in the elastic modulus. Second, it requires collecting a large number of data points per pixel in order to retrieve the material properties with reasonable accuracy. Those difficulties have set the motivation to develop nanomechanical spectroscopy methods based on the use of either amplitude [38] or frequency modulation AFM methods [39] . Here we develop a nanoscale microscopy method that enables the simultaneous mapping of the Young’s modulus, the viscous coefficient, the indentation and the topography of several polymer surfaces. The method combines bimodal excitation and detection for simultaneous mapping of several properties, frequency modulation feedbacks for sensitivity and fractional calculus for relating observables to nanomechanical properties. The validity of the method has been tested by using calibration samples and by comparing the experimental results with numerical simulations. This method requires four data points per pixel to provide a nanomechanical description of the surface (stiffness, viscosity, deformation and peak force). The above property speeds up data acquisition while minimizing the amount of data used in the measurements. In addition, the nanomechanical measurements are insensitive to the imaging parameters that prevent the cross-talk between topography and material properties. Bimodal AFM in frequency modulation The development of a bimodal nanomechanical spectroscopy for soft matter is divided into three major steps ( Fig. 1 ): first, the method to acquire several independent observables simultaneously ( Fig. 1b ); second, the feedback processes to control and stabilize the operation of the microscope ( Fig. 1c,d ); and third, the underlying theory that enables the transformation of observables into nanomechanical properties ( Fig. 1e,f ). The above steps should be compatible with a high data acquisition speed and the high spatial resolution of AFM. 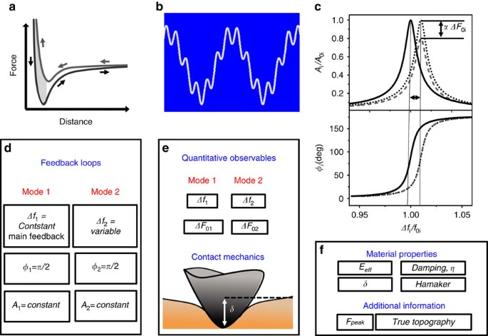Figure 1: Scheme of bimodal nanomechanical spectroscopy. (a) Scheme of a force curve. The shaded area indicates the dissipation introduced by repulsive interactions. The arrows indicate the direction of the tip motion. (b) Tip excitation in bimodal AFM. It has a large amplitude component tuned at the first flexural mode of the cantilever and a small component tuned at the second flexural frequency. (c) Scheme of the frequency shift, phase shift, amplitude reduction and correction in frequency modulation AFM. (d) Block diagram depicting the feedback controls in bimodal nanomechanical spectroscopy.(e) Scheme of the main observables and contact mechanics deformation. (f) Outcomes of the method. Figure 1: Scheme of bimodal nanomechanical spectroscopy. ( a ) Scheme of a force curve. The shaded area indicates the dissipation introduced by repulsive interactions. The arrows indicate the direction of the tip motion. ( b ) Tip excitation in bimodal AFM. It has a large amplitude component tuned at the first flexural mode of the cantilever and a small component tuned at the second flexural frequency. ( c ) Scheme of the frequency shift, phase shift, amplitude reduction and correction in frequency modulation AFM. ( d ) Block diagram depicting the feedback controls in bimodal nanomechanical spectroscopy. ( e ) Scheme of the main observables and contact mechanics deformation. ( f ) Outcomes of the method. Full size image Our method is based on the bimodal AFM scheme in which the first two flexural cantilever modes are excited by two external forces tuned at the free resonant frequencies of those modes [32] , [40] ( Fig. 1b ). The frequency shift of the first flexural mode Δ f 1 is kept at a fixed value during imaging while the oscillation amplitude is kept constant, A 1 =constant in the presence of dissipation by changing the excitation signal Δ F 01 . The changes in the frequency shift are followed by keeping the phase shift locked at 90° with phase-locked loops ( Fig. 1c ). On the second mode, the changes of the resonant frequency are recorded while the oscillation amplitude is kept constant ( A 2 =constant). The instrument has five different feedback loops for feedback control ( Fig. 1d ). Bimodal AFM allows for four independent observables without compromising the spatial resolution or the data acquisition speed. When used in this configuration with four additional feedback loops, these observables are Δ f i and Δ F 0 i ( i =1, 2). While the additional feedback loops do complicate the measurement, they have the advantage of giving us observables that can be related to parameters of the model through analytic expressions. The amplitude of the first mode A 1 is more than one order of magnitude larger than the amplitude of the second mode. Two things are gained by using this asymmetry. First, the operation of the microscope is stabilized by the first mode. Second, A 2 can be considered a small perturbation of the total amplitude ( A 1 + A 2 ), which facilitates the derivation of the analytical expressions. Theory of nanomechanical spectroscopy The transformation of experimental observables into nanomechanical properties is divided into two major steps. First, the theory that provides the analytical expressions that relate the experimental observables to the tip-surface forces. The second step involves the transformation of forces into material properties. This is accomplished by using suitable contact mechanics models. In bimodal frequency modulation AFM, the frequency shift of any mode is related to the force by [23] , [41] , [42] where f 0 i , k i and A i stand, respectively, for the resonant frequency in the absence of a force, the force constant and the amplitude of mode i (see Methods). The above Equation is a generalization of the expression used in conventional frequency modulation AFM for the fundamental mode [43] . The tip-surface force includes both conservative and dissipative interactions modeled, respectively, by the Hertz contact mechanics and a linear viscoelastic theory. Then the tip-surface force is expressed by where d is the instantaneous tip-sample distance, R is the tip radius, δ is the sample indentation ( δ = a 0 −d , with a 0 =0.165 nm) and η is the viscous coefficient. E eff is the effective Young’s modulus of the interface. As the probe Young’s modulus E tip is at least two orders of magnitude larger than those of the samples studied here E eff ~ E s . Long-range attractive forces and capillary forces have not been considered because the experiments are performed with sharp tips and under dry nitrogen environments. Under those conditions, the dominant forces are short-range repulsive (contact) forces. The combination ofEquations 1 and 2, the use of fractional calculus methods [42] , [44] , [45] and the bimodal scheme developed here enables the application of the following analytical expressions between the observables and the material properties, where F 0 i and ΔF 0 i are, respectively, the initial excitation force and the change in the excitation force needed to keep the A i constant. The indentation is calculated by Validation of the method The bimodal nanomechanical spectroscopy has an internal protocol that enables to select or disregard the experimental data. Equation (3) can be rewritten to show a linear relationship between Δ f 1 and Δ f 2 2 where d m is the closest distance between tip and sample (Methods). Consequently, only the data compatible with Equation (6) are used for the nanomechanical measurements. The presence of large adhesion forces and/or the use of a tip with an irregular geometry modify the relationship between the excited frequencies so that the above linear dependence is no longer observed. The above relationship is strictly valid for Hertz contact mechanics. Materials described with a different contact mechanics model will have a different relation between Δf 1 and Δf 2 2 . We have also deduced the expressions for van der Waals forces and Sneddon models. 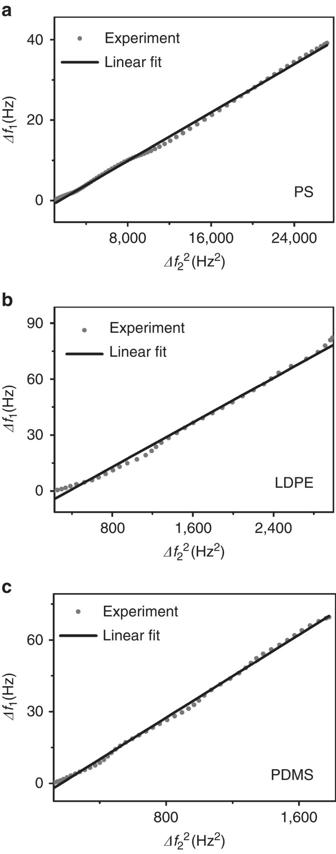Figure 2: Linear relationships between the 1st and 2nd flexural modes. (a) Polystyrene (~2.0 GPa). (b) Polyolefin elastomer (LDPE) (~0.1 GPa). (c) polydimethylsiloxane (~2.5 MPa). The experimental data should bear a linear relationship betweenΔf1andΔf22to apply the bimodal nanomechanical spectroscopy.A1=40 nm. Figure 2 shows the relationship between Δf 1 and Δf 2 2 obtained for three polymer surfaces with the Young’s modulus ( E s ) ranging from about 1 MPa to 3 GPa. The same cantilever-tip system has been used to get the data (SSS-NCL, Nanoworld). Figure 2: Linear relationships between the 1st and 2nd flexural modes. ( a ) Polystyrene (~2.0 GPa). ( b ) Polyolefin elastomer (LDPE) (~0.1 GPa). ( c ) polydimethylsiloxane (~2.5 MPa). The experimental data should bear a linear relationship between Δf 1 and Δf 2 2 to apply the bimodal nanomechanical spectroscopy. A 1 =40 nm. Full size image Probe calibration The present nanomechanical measurements imply the determination of several parameters of the microscope such as the force constants, quality factors of the excited modes and the tip’s radius. The force constants and quality factors are determined by using the thermal noise method [46] , [47] . Typical values for the experiments shown here are k 1 =20 N m −1 , k 2 =760 N m −1 ; Q 1 =300, Q 2 =500. The effective tip radius R is determined by reproducing the Young’s modulus of a polystyrene (PS) sample with a nominal value of 2.7 GPa. Calibration test A new method needs to reproduce the mechanical properties of some samples with well-known properties. We have recorded bimodal nanomechanical maps on a calibration sample made of circular regions of a polyolefin elastomer (LDPE) embedded in a matrix of PS. The above regions have nominal Young’s modulus of 100 MPa and 2.0 GPa. The Poisson’s ratio is 0.35 for LDPE and 0.34 for PS. In Fig. 3 we show the maps of the experimental observables and the materials property maps. Those maps together with the topography are taken simultaneously. The AFM image shows a series of circular regions with a diameter that varies between 1 and 2 μm surrounded by relatively flat regions. The AFM image and the nanomechanical maps have been taken by changing the set-point parameter of the main feedback seven times from Δf 1 =37 to 97 Hz (approximately every 450 nm along the y axis). This is reflected in the colour-coded maps of the observables Δf 1 , Δf 2 , ΔF 01 and ΔF 02 ( Fig. 3a–d ). The corresponding histograms show between seven and nine peaks ( Fig. 3e–h ). In the case of Δf 1 ( x , y ) the peaks are imposed by changing the main feedback value, while for the other maps the peaks reflect both the changes in the feedback and the changes of the nanomechanical response of the sample. For example, the Δf 2 ( x , y ) map shows nine peaks, seven coming from the PS regions and two from the elastomer. 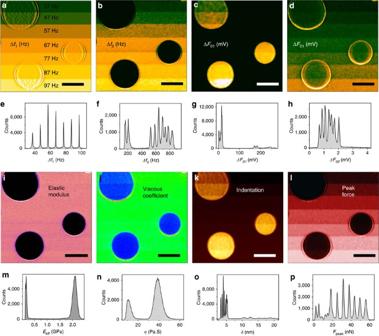Figure 3: Nanomechanical maps of a polymer blend. (a) Map ofΔf1(x,y). The image has been recorded by changing the main feedback approximately every 450 nm in the slow scanning direction (scale bar, 750 nm). (b) Map ofΔf2(x,y). The changes inΔf2reflect both the changes in the elastic response of the blend and the changes of the main feedback (scale bar, 750 nm). (c) Map ofΔF01(x,y). The map shows the changes in the driving force of mode 1 to compensate the instantaneous changes inA1while imaging (scale bar, 750 nm). (d) Map ofΔF02(x,y). The map shows the changes in the driving force of mode 2 to compensate the instantaneous changes inA2while imaging (scale bar, 750 nm). (e).Histogram ofΔf1obtained froma. (f) Histogram ofΔf2obtained fromb. (g) Histogram ofΔF01(x,y) obtained fromc.(h) Histogram ofΔF01(x,y) obtained fromd(i) Map of the elastic modulus across the surface. Two regions are observed. A softer region in the circles and a stiffer region in the rest of the surface. Those regions correspond, respectively, to the LDPE and PS (see histogram inm) (scale bar, 750 nm). (j) Map of the viscous coefficient. Two regions are observed. Lower damping (viscous) coefficients are found in the softer regions (LDPE) while the PS regions give higher damping coefficients (see histogram inn) (scale bar, 750 nm). (k) Map of the indentation. The indentation depends on both the elastic response and the set-point value (scale bar, 750 nm). (l) Map of the peak force (maximum force). It reproduces the trend observed in the indentation (scale bar, 750 nm). (m) Histogram of theEeffvalues. The values do not depend on the feedback parameters. (n) Histogram of viscous coefficient. The values do not depend on the feedback parameters. (o) Histogram of the indentation. (p) Histogram of peak force values. The data has been recorded in 2 minutes. Figure 3: Nanomechanical maps of a polymer blend. ( a ) Map of Δf 1 ( x , y ). The image has been recorded by changing the main feedback approximately every 450 nm in the slow scanning direction (scale bar, 750 nm). ( b ) Map of Δf 2 ( x , y ). The changes in Δf 2 reflect both the changes in the elastic response of the blend and the changes of the main feedback (scale bar, 750 nm). ( c ) Map of ΔF 01 ( x , y ). The map shows the changes in the driving force of mode 1 to compensate the instantaneous changes in A 1 while imaging (scale bar, 750 nm). ( d ) Map of ΔF 02 ( x , y ). The map shows the changes in the driving force of mode 2 to compensate the instantaneous changes in A 2 while imaging (scale bar, 750 nm). ( e ).Histogram of Δf 1 obtained from a . ( f ) Histogram of Δf 2 obtained from b . ( g ) Histogram of ΔF 01 ( x , y ) obtained from c. ( h ) Histogram of ΔF 01 ( x , y ) obtained from d ( i ) Map of the elastic modulus across the surface. Two regions are observed. A softer region in the circles and a stiffer region in the rest of the surface. Those regions correspond, respectively, to the LDPE and PS (see histogram in m ) (scale bar, 750 nm). ( j ) Map of the viscous coefficient. Two regions are observed. Lower damping (viscous) coefficients are found in the softer regions (LDPE) while the PS regions give higher damping coefficients (see histogram in n ) (scale bar, 750 nm). ( k ) Map of the indentation. The indentation depends on both the elastic response and the set-point value (scale bar, 750 nm). ( l ) Map of the peak force (maximum force). It reproduces the trend observed in the indentation (scale bar, 750 nm). ( m ) Histogram of the E eff values. The values do not depend on the feedback parameters. ( n ) Histogram of viscous coefficient. The values do not depend on the feedback parameters. ( o ) Histogram of the indentation. ( p ) Histogram of peak force values. The data has been recorded in 2 minutes. Full size image The maps of the material properties ( Fig. 3i–l ) are obtained by processing the data of Fig. 3a–d with the equations introduced above. The elastic modulus and viscosity coefficient maps show the existence of two regions that match the morphology of the polymer blend ( Fig. 3i,j ). The circular regions show a Young’s modulus of 168±30 MPa, while the surrounding matrix has a mean value of 2.1±0.1 GPa ( Fig. 3m ). Those values coincide or are very close to the expected values for this material (100 MPa and 2 GPa, respectively). The viscosity (damping) maps taken at 1.8 MHz show two mean values, one centred at 11±4 Pa s (LDPE) and the other at 39±8 Pa s (PS) ( Fig. 3n ). The same maps taken at the frequency of the first mode (292,214 Hz) give, respectively, 40 and 120 Pa s. The above nanomechanical measurements do not depend on the set-point values. This can be considered as an indication of the absence of artifacts in the measurements. The above maps have been acquired in less than 2 min. The indentation map depends on the frequency set-point value because this controls the maximum force (peak force) exerted on the sample. It also depends on the local compliance of the sample. This is reflected in the corresponding histogram ( Fig. 3o ) where the observed peaks are grouped in two different regions one corresponding to the PS and the other to the LDPE regions. In the relative stiff regions (PS) the peaks are tightly found between 1 and 5 nm while for the softer regions (LDPE) the peaks are scattered between 10 and 20 nm. The peaks obtained in the LDPE regions are smaller because the area of the LDPE regions is smaller than area of the PS. The AFM topography images cannot be considered as real topography especially while imaging soft matter [48] , [49] . This is reflected in the dependence of the indentation of the set-point frequency shift ( Fig. 3k,o ). However, the bimodal nanomechanical spectroscopy offers a method to reconstruct the real topography of polymer surfaces, and in particular, the polymer blend by combining the apparent topography with the indentation map. The value of the peak force depends on both the compliance of the surface and the set-point frequency shift. Seven peak force values are found in the PS regions; they range between 18 and 56 nN ( Fig. 3p ). In the LDPE regions, we only distinguish five peaks with forces ranging between 2 and 14.5 nN. To illustrate the sensitivity to distinguish between different soft materials we have imaged two Polydimethylsiloxane (PDMS) surfaces, one characterized with a nominal Young’s modulus of 2.5 MPa and the other with 3.5 MPa. The measurements have been performed with the same tip and under the same experimental conditions. The AFM topography shows a granular structure with a grain diameter in the 10- to 25-nm range ( Fig. 4a,b ). The granularity of the surface is preserved both in the elastic and the viscous coefficient maps. We notice that for the stiffer PDMS (3.5 MPa), the spatial resolution observed in the image matches the theoretical maximum for a tip of 2 nm and a peak force of 1 nN. The nanomechanical maps are shown in Fig. 4c–f . The values of the E eff and η are shown in the histograms ( Fig. 4g,h ). The distribution shows a mean value of 3.2±0.1 MPa and 7.8±0.1 Pa s (at 152,997 Hz). The roughness of the surface implies that the tip might interact with different regions of the PDMS at the same time. This gives rise to the local changes observed in the maps. 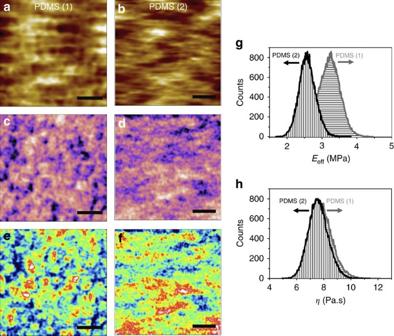Figure 4: Nanomechanical maps of soft polymers. The same tip is used to map PDMS samples of different elastic moduli. (a) Topography (apparent) of a PDMS sample of a nominalEPDMS1=3.5 MPa (scale bar, 50 nm). (b) Topography (apparent) of a PDMS sample of a nominalEPDMS2=2.5 MPa (scale bar, 50 nm). (c) Map of the elastic modulus of PDMS1 (scale bar, 50 nm). (d) Map of the elastic modulus of PDMS2 (scale bar, 50 nm). (e) Map of the viscosity of PDMS1 (scale bar, 50 nm). (f) Map of the viscosity of PDMS2 (scale bar, 50 nm). (g) Histogram of the elastic modulus. (h) Histogram of viscous coefficient. Figure 4: Nanomechanical maps of soft polymers. The same tip is used to map PDMS samples of different elastic moduli. ( a ) Topography (apparent) of a PDMS sample of a nominal E PDMS1 =3.5 MPa (scale bar, 50 nm). ( b ) Topography (apparent) of a PDMS sample of a nominal E PDMS2 =2.5 MPa (scale bar, 50 nm). ( c ) Map of the elastic modulus of PDMS1 (scale bar, 50 nm). ( d ) Map of the elastic modulus of PDMS2 (scale bar, 50 nm). ( e ) Map of the viscosity of PDMS1 (scale bar, 50 nm). ( f ) Map of the viscosity of PDMS2 (scale bar, 50 nm). ( g ) Histogram of the elastic modulus. ( h ) Histogram of viscous coefficient. Full size image The ability of bimodal spectroscopy to distinguish between the two PDMS surfaces and to provide values of the elastic modulus very close to the nominal values (2.1±0.1 versus 2.5 MPa and 3.2±0.1 versus 3.5 MPa) gives an indication of the accuracy and sensitivity of the method. The damping coefficients measured at the frequency of the first mode (152,860 Hz) give rather similar values of 7.6 Pa s for PDMS2 and 7.8 Pa s for PDMS1. The present method does not interfere with the standard configuration of frequency modulation AFM; as a consequence the spatial resolution remains unaffected. To illustrate the spatial resolution we have imaged a surface of a block copolymer polystyrene-b-poly(methyl methacrylate) (PS-b-PMMA) thin film. The diblock copolymer forms ordered structures alternating PS and PMMA domains. The elastic modulus and indentation maps ( Fig. 5a,b ) show the presence of either flat or vertical PMMA cylinders (stiffer domains). The average diameter of the PMMA cylinders in both maps is of 17 nm. A cross-section taken from the indentation map ( Fig. 5c ) demonstrates a lateral resolution in the sub-17-nm range. Identical resolution is obtained in the viscous coefficient map. 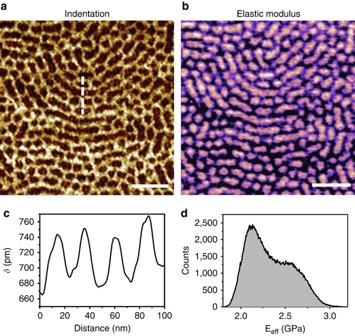Figure 5: Spatial resolution in elastic modulus map. (a) Indentation map in a block copolymer (PS-b-PMMA) thin film (scale bar, 100 nm). (b) Map of the elastic modulus of PS-b-PMMA (scale bar, 100 nm). (c) Cross-section along the dashed line shown ina. (d) Histogram of the elastic modulus obtained fromb. Figure 5: Spatial resolution in elastic modulus map. ( a ) Indentation map in a block copolymer (PS-b-PMMA) thin film (scale bar, 100 nm). ( b ) Map of the elastic modulus of PS-b-PMMA (scale bar, 100 nm). ( c ) Cross-section along the dashed line shown in a . ( d ) Histogram of the elastic modulus obtained from b . Full size image The histograms obtained from Fig. 5b show the presence of two peaks ( Fig. 5d ): a dominant peak centred at 2.11 GPa that comes from the PS regions and another shoulder-like peak centred at 2.6 GPa that comes from the PMMA regions. Notice that the contrast in the indentation and Young’s modulus maps is inverted. The indentation is smaller in the PMMA domains than in the PS regions because the Young’s modulus of PMMA is higher than that of PS. The bimodal nanomechanical spectroscopy enables the measurement of several mechanical properties with nanoscale spatial resolution. Elastic and dissipative parameters of heterogeneous surfaces have been measured simultaneously with the apparent topography and the indentation. The method also provides for each point of the surface the maximum value of the force exerted on it. Several features set this method apart from other force microscopy proposals. This method requires four data points per pixel to provide a nanomechanical description of the surface (stiffness, viscosity, deformation and peak force). The above feature speeds up data acquisition and minimizes the amount of data processed by the instrument. The same cantilever-tip system can be used to measure elastic properties covering a near four order of magnitude range. We have explored materials from 1 MPa to ~3 GPa. The theory behind this nanomechanical spectroscopy enables to determine beforehand the accuracy and/or suitability of a given measurement. In addition, the nanomechanical measurements are insensitive to the imaging parameters, which prevent the cross-talk between topography and material properties. Finally, this nanomechanical spectroscopy is compatible with standard microcantilevers and dynamic force microscopy configurations. Cantilevers The data reported here have been taken with two cantilevers. Cantilever 1 (SSS-NCL SuperSharpSilicon cantilever, Nanoworld, Germany) is characterized by f 01 =152,860 Hz, k 1 =22 N m −1 , Q 1 =366, f 02 =950,533 Hz, k 2 =850 N m −1 , Q 2 =474. Cantilever 2 (NCHV, Bruker) is characterized by f 01 =292,214 Hz, k 1 =9.2 N m −1 , Q 1 =434, f 02 =1.8343 MHz, k 2 =362 N m −1 , Q 2 =620. The optical lever sensitivity of the first mode is determined by acquiring a force curve on a stiff surface (mica). The force constant of the first mode is determined by using the thermal method, while the force constant of the second mode is determined from the theoretical relationships between the force constant of the first and second modes [15] . Polymer samples Three polymer samples have been used. A polymer blend made of PS regions ( E PS ≈2.0 GPa) and polyolefin elastomer (ethylene-octene copolymer) (LDPE) ( E LDPE ≈0.1 GPa) has been used. In both cases nominal values. We have also used two types of PDMS surfaces, with macroscopic elastic moduli of 3.5 and 2.5 MPa. Those samples were acquired from Bruker AFM probes. To estimate the lateral resolution we have used a block copolymer PS-b-PMMA layer. The length of the PS-b-PMMA is 34 nm and the layer thickness (average value) is ~50 nm. The polymer layer was prepared as described by Oria et al . [50] . AFM measurements The codes developed here have been implemented into a commercial AFM (Cypher, Asylum Research). The AFM data have been acquired at a scan frequency for the fast x axis of 2 Hz. Typical values for the first and second amplitudes were, respectively, 15–90 and 0.3–0.6 nm. The experiments have been performed in air. Bimodal nanomechanical spectroscopy equations The transition from Equations (1) and (2) to Equations (3) and (4) requires a series of intermediate steps. where z c is the mean tip-surface separation and d m is the closest distance between tip and sample in an oscillation cycle, On the other hand, because A 1 >>A 2 the frequency shifts depend on the mode [42] . In particular, modes 1 and 2 are expressed, respectively, as where the fractional integrals and derivatives are calculated by using the Riemann–Liouville fractional calculus [51] which leads to a relationship between the frequency shifts and the effective Young’s modulus and the indentation, where for d m ≤0, δ = a 0 −d m with a 0 =0.165 nm. Similarly, the viscosity is related to the experimental observables by where We have used the following two main hypotheses to deduce the Equations (9) and (10): (a) A 1 is larger than the typical length of scale of the interaction force and (b) A 2 should satisfy The implications of the above hypothesis can be checked experimentally by recovering the force with Sader method [44] and comparing its numerical half integral with the results given by Equation (9) and its numerical half derivative with the results given by Equation (10). How to cite this article: Herruzo, E. T. et al . Fast nanomechanical spectroscopy of soft matter. Nat. Commun. 5:3126 doi: 10.1038/ncomms4126 (2014).